Drebrin-like protein DBN-1 is a sarcomere component that stabilizes actin filaments during muscle contraction Actin filament organization and stability in the sarcomeres of muscle cells are critical for force generation. Here we identify and functionally characterize a Caenorhabditis elegans drebrin-like protein DBN-1 as a novel constituent of the muscle contraction machinery. In vitro , DBN-1 exhibits actin filament binding and bundling activity. In vivo , DBN-1 is expressed in body wall muscles of C. elegans . During the muscle contraction cycle, DBN-1 alternates location between myosin- and actin-rich regions of the sarcomere. In contracted muscle, DBN-1 is accumulated at I-bands where it likely regulates proper spacing of α-actinin and tropomyosin and protects actin filaments from the interaction with ADF/cofilin. DBN-1 loss of function results in the partial depolymerization of F-actin during muscle contraction. Taken together, our data show that DBN-1 organizes the muscle contractile apparatus maintaining the spatial relationship between actin-binding proteins such as α-actinin, tropomyosin and ADF/cofilin and possibly strengthening actin filaments by bundling. Sarcomeres are the fundamental morphological and functional units of myofibrils in striated muscle cells. During muscle contraction, sarcomeres undergo a reversible shortening driven by central, bipolar myosin filaments pulling on actin filaments that are attached at the sarcomere boundaries, thus contracting the sarcomeres. This process is normally reversible, that is, during muscle relaxation the myosin filaments detach from actin filaments allowing the sarcomeres to return to their pre-contraction state. The correct timing and coordination of contraction cycles is mediated by a fascinating orchestration of what one could call a ‘functional cloud’ of numerous structural and regulatory proteins. This general scheme of a cloud of different proteins involved in regulation of function is observed in many other cellular machineries, such as the centromeres [1] , [2] , centrosomes [3] , [4] , focal adhesion complexes [5] , [6] or the plus ends of microtubules [7] . In the case of the highly regulated muscle machinery, new players still emerge, contributing to an ever more precise picture of muscle function. One of the best experimental model organisms to study muscle contraction at the sarcomere level in live animals is the small nematode C. elegans . Extensive conservation of the basic protein components within the sarcomere structure between C. elegans and human makes the body-wall muscle system suitable to investigate the genetic and molecular basis of human muscle diseases [8] , [9] . A typical striated body-wall muscle cell of the nematode has three parts: the contractile myofilament lattice, a non-contractile muscle belly containing the nucleus and intracellular organelles, and the muscle arms, slender processes that extend to either ventral or dorsal nerve cords or the nerve ring. The myofilament lattice is restricted to a narrow 1.5-μm thick layer at the outer side of the cell, adjoining the cell membrane. The actin filaments are attached to the dense bodies (the analogues of mammalian Z-discs), and the myosin filaments are organized around the M-lines. Striation of body wall muscle cells is visible due to the alternation of myosin-filament-containing (A-band) and only actin-filament-containing (I-band) regions. In contrast to mammalian striated muscle, sarcomeres in C. elegans are oriented not at 90° but at a sharp angle of only 5.9° to the muscle long axis [10] , [11] . Dense bodies and M-lines are anchored to the muscle cell membrane and the extracellular matrix, which, in turn, are attached to the hypodermis and cuticle. This allows the transmission of contractile force directly from actin filaments to the cuticle, which then drives movement of the whole animal. To produce contractile force, actin filaments inside a sarcomere must be properly anchored, positioned and stabilized by means of specific actin-binding proteins. The protein α-actinin connects actin filaments to the Z-disk and the dense body [12] , [13] . Tropomyosin is attached to actin filaments as a structural scaffold in the overlap region with myosin, between I-bands and M-lines [14] , [15] and inhibits spontaneous actin polymerization [16] , [17] and depolymerization from the pointed ends [18] , [19] . Together with troponin, tropomyosin regulates acto–myosin interactions [20] . Actin filament dynamics are further regulated by members of the actin-depolymerizing factor homology (ADF-H) family, which is subdivided into three structurally distinct classes: ADF/cofilins, twinfilins and drebrins/Abp1s [21] . The best-described protein of the first class in C. elegans is the ADF/cofilin homologue UNC-60B. Inside the sarcomere, this protein is localized to the I-band and enhances actin-filament turnover by accelerating the rate of depolymerization at the pointed ends and by severing filaments [22] , [14] . Mutations in the unc-60B gene result in the formation of highly disorganized sarcomeres and the appearance of large aggregates of actin at the lateral ends of body-wall muscle cells [23] . The second class member twinfilin is expressed in mammalian skeletal and heart muscles [24] . In vitro , twinfilin binds to actin monomers and inhibits actin polymerization [25] , [26] . While the players of the third class, drebrin 1 (DBN1) and drebrin-like protein (DBNL; also known as Abp1, SH3P7 and HIP-55) have been associated with the function of neurological and immunological synapses [27] , [28] , [29] , [30] , their role in the sarcomere was unknown. Notably, in C2C12 myoblasts, expression of drebrin is induced during differentiation and is essential for myotube formation [31] . Mutation of mAbp1 in mice results in various organ abnormalities, including development of hypertrophic cardiomyopathy [32] . The existence of an open reading frame in the C. elegans genome that encodes an uncharacterized protein related to Abp1 was first mentioned in ref. 33 . We here report on the function of this protein, encoded by the K08E3.4 gene, and name it DBN-1 (for DreBriN 1/DreBriN-like homologue). We show that DBN-1 is expressed in body-wall muscle cells and that it is essential for sarcomere organization. Our functional analysis revealed that DBN-1 stabilizes actin filaments during muscle contraction and directs the proper localization of ADF/cofilin, tropomyosin and α-actinin in the myofilament lattice. DBN-1 is a C. elegans homologue of mAbp1 and drebrin 1 First we compared the protein sequence of C. elegans DBN-1, encoded by the K08E3.4 gene, with its mammalian homologues drebrin and mAbp1. DBN-1 contains an ADF-H domain, a coiled-coil region, a proline-rich region and an SH3 domain ( Fig. 1a ). The N-terminal ADF-H domain of DBN-1 has a strong sequence similarity to the corresponding regions of all class members. The region following the ADF-H domain contains three isolated coiled-coil domains, in contrast to one coiled-coil domain in the structures of drebrin and mAbp1 ( http://embnet.vital-it.ch/software/COILS_form.html ). The proline-rich region of DBN-1 is more similar to the corresponding region of drebrin 1 than to that of mAbp1. Finally, the C-terminal SH3 domain of DBN-1 has 59% identity to the SH3 domain of mAbp1, whereas drebrin does not contain it [33] . Overall, DBN-1 thus appears to be a canonical member of the ADF-H family, drebrin/mAbp1 class of actin-binding proteins, albeit with interesting differences to its relatives. 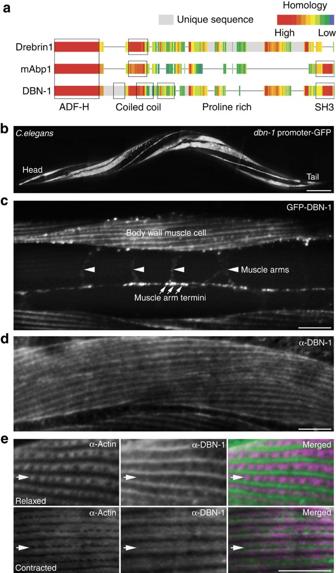Figure 1: Localization of DBN-1 inC. elegans. (a) Comparative domain alignment ofMus musculusdrebrin1 (NCBI accession number NP_001170842.1), mAbp1 (NP_001139780.1) and DBN-1 (NP_499840.1). Protein sequence alignment was performed using the T-coffee program (http://www.tcoffee.org/) followed by assembly in Adobe Photoshop CS5.1. DBN-1 contains an N-terminal ADF-H domain, three coiled-coil domains, a proline-rich domain and a C-terminal SH3 domain. Colour scale: red=100% to blue=0% identity; grey colour indicates unique sequence. (b) TransgenicC. elegansexpressing adbn-1 promoter-GFPreporter construct. Thedbn-1promoter drives GFP expression in body wall muscle cells. Scale bar, 50 μm. (c) Expression of GFP-DBN-1 in body wall muscles driven by the muscle-specifichim-4promoter. GFP-DBN-1 is localized mainly to the myofilament lattice and in cluster-like structures at muscle arm termini. Scale bar, 10 μm. (d) Distribution of endogenous DBN-1 in body wall muscle cells revealed by indirect immunofluorescence with anti-DBN-1 antibodies. Scale bar, 10 μm. (e) Localization of endogenous DBN-1 relative to endogenous actin in relaxed and contracted muscles. Scale bar, 10 μm. Figure 1: Localization of DBN-1 in C. elegans . ( a ) Comparative domain alignment of Mus musculus drebrin1 (NCBI accession number NP_001170842.1), mAbp1 (NP_001139780.1) and DBN-1 (NP_499840.1). Protein sequence alignment was performed using the T-coffee program ( http://www.tcoffee.org/ ) followed by assembly in Adobe Photoshop CS5.1. DBN-1 contains an N-terminal ADF-H domain, three coiled-coil domains, a proline-rich domain and a C-terminal SH3 domain. Colour scale: red=100% to blue=0% identity; grey colour indicates unique sequence. ( b ) Transgenic C. elegans expressing a dbn-1 promoter-GFP reporter construct. The dbn-1 promoter drives GFP expression in body wall muscle cells. Scale bar, 50 μm. ( c ) Expression of GFP-DBN-1 in body wall muscles driven by the muscle-specific him-4 promoter. GFP-DBN-1 is localized mainly to the myofilament lattice and in cluster-like structures at muscle arm termini. Scale bar, 10 μm. ( d ) Distribution of endogenous DBN-1 in body wall muscle cells revealed by indirect immunofluorescence with anti-DBN-1 antibodies. Scale bar, 10 μm. ( e ) Localization of endogenous DBN-1 relative to endogenous actin in relaxed and contracted muscles. Scale bar, 10 μm. Full size image DBN-1 is expressed in body-wall muscles Next we analysed the tissue expression pattern of DBN-1 to close in on its function. We generated transgenic C. elegans strains, in which green fluorescent protein (GFP) expression was driven by the 2,003 bp dbn-1 promoter. In all eight lines obtained, a GFP signal was detected in body-wall muscle cells ( Fig. 1b ). This result points to a primary function of DBN-1 in striated muscles. To analyse the distribution of DBN-1 in live striated muscle cells, we expressed GFP-tagged DBN-1 under the control of the body wall muscle-specific him-4 promoter. In live C. elegans , DBN-1 was mostly localized in a striated pattern coinciding with sarcomeres, within the cytosol and furthermore concentrated at muscle arm termini, which represent the postsynaptic sites of neuromuscular junctions ( Fig. 1c ). To confirm the subcellular localization of endogenous DBN-1, we produced rabbit polyclonal antibodies against the full-length DBN-1 and performed indirect immunostaining of whole worms. The endogenous DBN-1 localized within body wall muscle cells in a striated pattern ( Fig. 1d ). At closer inspection, DBN-1 revealed striking features in localization with respect to actin filaments. In relaxed muscles, in which actin was concentrated near dense bodies, DBN-1 localized at M-lines ( Fig. 1e ). In contracted muscles, where actin occupied a much broader space, extending to M-lines, DBN-1 co-localized with actin filaments at their distal parts close to dense bodies ( Fig. 1e ). DBN-1 localization changes dynamically during contraction To demonstrate that the targeting of DBN-1 to different parts of the sarcomere is indeed dependent on the muscle contraction state, we monitored GFP-DBN-1 dynamics in contracting muscles of live non-anaesthetized nematodes. Fluorescence time-lapse microscopy revealed drastic changes in localization of GFP-DBN-1 inside the sarcomere during contraction cycles ( Fig. 2b,c ; Supplementary Movie 1 ). In relaxed muscle, GFP-DBN-1 localized in a striated pattern of alternating dashed and continuous lines. During muscle contraction, dashed lines transformed into continuous lines, while the initially continuous lines disappeared. We found that the continuous lines in the relaxed muscle coincided with M-lines, and that the dashed patterns between them coincided with dense bodies. The continuous lines appearing at contraction are in the I-bands ( Fig. 3 ). This change of localization of DBN-1 was reversible and persisted over multiple contraction cycles. We quantified the changing patterns by Fourier analysis ( Fig. 2d ). A comparison of Fourier transforms of images of relaxed and contracted muscles shows a shift of the line spacing from 0.86 μm in the relaxed state to 1.65 μm in the contracted state, that is, an almost exact doubling of the distance, corresponding to the disappearance of the labelling at the M-lines. A further intriguing result of this analysis is that contraction in the C. elegans body wall muscle mainly results in an increase of the angle between sarcomeres and the muscle long axis leaving the distance between I-bands largely unaffected. This makes functional sense since in this manner sarcomere contraction is translated into shortening of the muscle long axis without inefficient contraction normal to the muscle long axis. 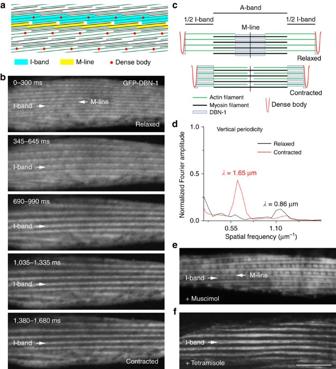Figure 2: Localization of DBN-1 in liveC. elegansduring muscle contraction. (a) Schematic representation of the sarcomere lattice in aC. elegansbody wall muscle cell. The sarcomeres are oriented at an angle of 5.9° to the muscle long axis. (b) Time series showing dynamics of GFP-DBN-1 distribution in contracting body wall muscle ofC. elegans. (c) Schematic localization of DBN-1 in the sarcomere in the relaxed and contracted states. (d) Spatial frequency profiles of GFP-DBN-1 patterns in the relaxed (black) and contracted (red) muscle shown inb. Spatial periods corresponding to the FFT peaks are indicated. (e) Localization of GFP-DBN-1 in body wall muscle after treatment with 10 mM muscimol. (f) Localization of GFP-DBN-1 in body wall muscle after treatment with 5 mM tetramisole. Scale bar, 10 μm. Figure 2: Localization of DBN-1 in live C. elegans during muscle contraction. ( a ) Schematic representation of the sarcomere lattice in a C. elegans body wall muscle cell. The sarcomeres are oriented at an angle of 5.9° to the muscle long axis. ( b ) Time series showing dynamics of GFP-DBN-1 distribution in contracting body wall muscle of C. elegans . ( c ) Schematic localization of DBN-1 in the sarcomere in the relaxed and contracted states. ( d ) Spatial frequency profiles of GFP-DBN-1 patterns in the relaxed (black) and contracted (red) muscle shown in b . Spatial periods corresponding to the FFT peaks are indicated. ( e ) Localization of GFP-DBN-1 in body wall muscle after treatment with 10 mM muscimol. ( f ) Localization of GFP-DBN-1 in body wall muscle after treatment with 5 mM tetramisole. Scale bar, 10 μm. 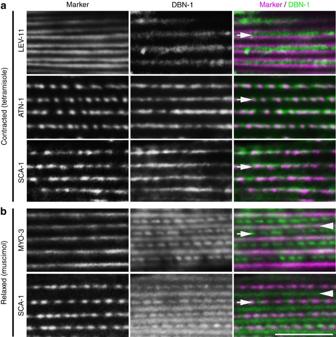Figure 3: Localization of DBN-1 with respect to other muscle proteins. (a) Body wall muscle cells of live young adult wild-type transgenicC. elegansparalysed in the contracted state by treatment with 5 mM tetramisole. Localization of GFP-LEV-11 and mCherry-DBN-1; mCherry-ATN-1 and GFP-DBN-1; mCherry-SCA-1 and GFP-DBN-1. (b) Body wall muscle cells of live young adult wild-type transgenicC. elegansparalysed in the relaxed state by treatment with 10 mM muscimol. Localization of mCherry-MYO-3 and GFP-DBN-1; mCherry-SCA-1 and GFP-DBN-1. Arrows indicate I-bands, arrowheads indicate M-lines. Scale bar, 10 μm. Full size image Figure 3: Localization of DBN-1 with respect to other muscle proteins. ( a ) Body wall muscle cells of live young adult wild-type transgenic C. elegans paralysed in the contracted state by treatment with 5 mM tetramisole. Localization of GFP-LEV-11 and mCherry-DBN-1; mCherry-ATN-1 and GFP-DBN-1; mCherry-SCA-1 and GFP-DBN-1. ( b ) Body wall muscle cells of live young adult wild-type transgenic C. elegans paralysed in the relaxed state by treatment with 10 mM muscimol. Localization of mCherry-MYO-3 and GFP-DBN-1; mCherry-SCA-1 and GFP-DBN-1. Arrows indicate I-bands, arrowheads indicate M-lines. Scale bar, 10 μm. Full size image To confirm our observations, we trapped muscles in either relaxed or contracted states by drug treatment: relaxing the muscle with the γ-aminobutyric acid receptor agonist muscimol (10 mM) or, alternatively, inducing persistent muscle contraction with the acetylcholine receptor agonist tetramisole (5 mM). Consistent with the observations in active muscle, in chemically relaxed body wall muscle cells GFP-DBN-1 localized at M-lines and at dense bodies ( Fig. 2e ; Fig. 3b ). In contrast, in chemically contracted muscle cells, DBN-1 accumulated at I-bands ( Fig. 2f ; Fig. 3a ). Thus, DBN-1 function in muscle evidently involves the shuttling between myosin- and actin-rich regions of the sarcomere during contraction. Localization of DBN-1 with respect to other muscle proteins The dynamic localization of DBN-1 in the sarcomere is likely to be coordinated with movements of other sarcomere components. To visualize such coordination in the ‘functional cloud’ within the sarcomere, we generated transgenic worms co-expressing fluorescently labelled DBN-1 together with several other sarcomere markers: α-actinin (ATN-1), tropomyosin (LEV-11), sarco–endoplasmic reticulum Ca 2+ -transport ATPase (SCA-1) and myosin heavy chain A (MYO-3). In body wall muscles contracted by tetramisole treatment, DBN-1 localized to I-bands, partially overlapping with ATN-1, but clearly demarcated from tropomyosin, which was located at the sides of I-bands ( Fig. 3a ). In muscimol-relaxed body wall muscle cells, DBN-1 localized to myosin filaments labelled with mCherry-MYO-3 and in a dashed pattern between them, where it was associated with the sarcoplasmic reticulum marker mCherry-SCA-1 ( Fig. 3b ). Interestingly, DBN-1 accompanied SCA-1 in both the contracted and relaxed state of muscles ( Fig. 3a,b ). DBN-1 interacts with F-actin in vivo Since DBN-1 is a member of the drebrin/Abp1 class of actin-binding proteins, we analysed its interaction with actin in vivo . If DBN-1 binds to actin, then changes of the polymerization state of actin should influence DBN-1 localization, and vice versa. We analysed the effect of actin depolymerization on the distribution of DBN-1 in cultured C. elegans muscle cells. In intact cells, GFP-DBN-1 was localized in the cytosol and at distinct sites of the plasma membrane, such as peripheral ruffles and endings of protrusion tips ( Fig. 4a , left). After treatment of these cells with 10 mM latrunculin A, the membrane pool of GFP-DBN-1 was immediately redistributed into the cytosol ( Fig. 4a , right). This shows that DBN-1 localization is highly sensitive to the actin polymerization state. To validate the interaction of DBN-1 and actin in vivo , we performed bimolecular fluorescence complementation (BiFC) assays. DBN-1 fused with the C-terminal part of Venus (VC155) was co-expressed with ACT-2 fused with the N-terminal part of Venus (VN155) in COS-7 cells under the control of the cytomegalovirus (CMV) promoter. A fluorescent BiFC signal, resulting from the formation of a macromolecular complex, was detected at peripheral ruffles of COS-7 cells ( Fig. 4b ). Together, these results indicate that DBN-1 can form functional macromolecular complexes with F-actin in vivo. 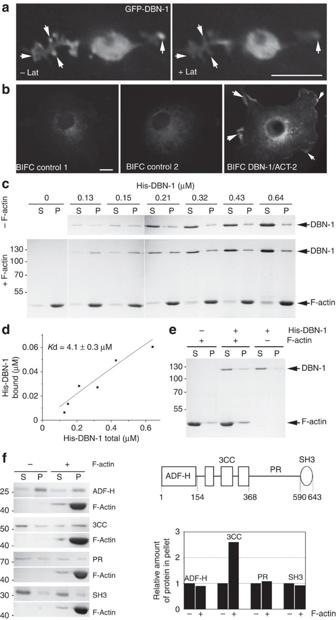Figure 4: DBN-1 interaction with F-actinin vivoandin vitro. (a) Live culturedC. elegansmuscle cell expressing GFP-DBN-1 before (left) and after (right) latrunculin A treatment. Scale bar, 10 μm. (b) Subcellular localization of the BiFC DBN-1-ACT-2 complex in COS-7 cells. Cos-7 cells were transfected with VN155-ACT-2 and VC155 alone (control 1); VC155-DBN-1 and VN155 alone (control 2) or VN155-ACT-2 and VC155-DBN-1 (BiFC). Arrows indicate localization of BiFC signal at peripheral ruffles of COS-7 cells. Scale bar, 10 μm. (c) Binding of DBN-1 to actin filamentsin vitro. Various concentrations of His-DBN-1 (as indicated) were incubated without or with F-actin (0.7 μM) for 1 h at room temperature, centrifuged at 100,000g, and the supernatants (S) and pellets (P) were analysed by SDS–polyacrylamide gel electrophoresis (SDS–PAGE). Molecular mass markers in kDa are indicated on the left. The actin-binding assay was performed three times with similar results. (d) The concentrations of His-DBN-1 bound to F-actin are plotted against the concentrations of total DBN-1 to determine theKdin actin-binding assays.Kdvalues represent mean with s.d. (e) Actin-bundling assay. F-actin alone, F-actin (1.4 μM) and His-DBN-1 (0.21 μM), or His-DBN-1 alone was incubated for 1 h at room temperature, centrifuged at 10,000g, and the supernatants (S) and pellets (P) were analysed by SDS–PAGE. (f) Actin-binding assays with GST-fusion ADF-H (aa 1–154), coiled-coil (3CC; aa154–368), proline-rich (PR; aa 369–590) and SH3 (aa 590–643) domains of DBN-1. Schematic representation of DBN-1 domains. Relative amount of GST-fusion proteins in the pellets without or with F-actin added in the reaction. Figure 4: DBN-1 interaction with F-actin in vivo and in vitro . ( a ) Live cultured C. elegans muscle cell expressing GFP-DBN-1 before (left) and after (right) latrunculin A treatment. Scale bar, 10 μm. ( b ) Subcellular localization of the BiFC DBN-1-ACT-2 complex in COS-7 cells. Cos-7 cells were transfected with VN155-ACT-2 and VC155 alone (control 1); VC155-DBN-1 and VN155 alone (control 2) or VN155-ACT-2 and VC155-DBN-1 (BiFC). Arrows indicate localization of BiFC signal at peripheral ruffles of COS-7 cells. Scale bar, 10 μm. ( c ) Binding of DBN-1 to actin filaments in vitro . Various concentrations of His-DBN-1 (as indicated) were incubated without or with F-actin (0.7 μM) for 1 h at room temperature, centrifuged at 100,000 g , and the supernatants (S) and pellets (P) were analysed by SDS–polyacrylamide gel electrophoresis (SDS–PAGE). Molecular mass markers in kDa are indicated on the left. The actin-binding assay was performed three times with similar results. ( d ) The concentrations of His-DBN-1 bound to F-actin are plotted against the concentrations of total DBN-1 to determine the K d in actin-binding assays. K d values represent mean with s.d. ( e ) Actin-bundling assay. F-actin alone, F-actin (1.4 μM) and His-DBN-1 (0.21 μM), or His-DBN-1 alone was incubated for 1 h at room temperature, centrifuged at 10,000 g , and the supernatants (S) and pellets (P) were analysed by SDS–PAGE. ( f ) Actin-binding assays with GST-fusion ADF-H (aa 1–154), coiled-coil (3CC; aa154–368), proline-rich (PR; aa 369–590) and SH3 (aa 590–643) domains of DBN-1. Schematic representation of DBN-1 domains. Relative amount of GST-fusion proteins in the pellets without or with F-actin added in the reaction. Full size image DBN-1 binds and bundles F-actin in vitro It remained to be tested whether DBN-1 binds to actin directly. For this, we performed an in vitro actin co-sedimentation assay. Recombinant His-fusion full-length DBN-1 was incubated with F-actin, centrifuged at high speed and analysed by SDS–polyacrylamide gel electrophoresis (SDS–PAGE). The actin-binding assay revealed that DBN-1 binds to actin filaments with a moderate affinity ( K d =4.1±0.3 μM) in a concentration-dependent manner ( Fig. 4c,d ). The binding of His-DBN-1 to F-actin saturated at a molar ratio of 0.054±0.001. This suggests that 1 molecule of His-DBN-1 can bind to approximately 18–19 molecules of F-actin, which may be a result of actin bundling that limits the available binding sites. We further examined the ability of DBN-1 to bundle F-actin by exploiting the fact that single actin filaments do not sediment at low centrifugation forces. After low-speed centrifugation, most of the F-actin in a control experiment was still present in the supernatant, whereas a significant amount of F-actin was pelleted after incubation with His-DBN-1 ( Fig. 4e ). This data confirms that, on top of its actin-binding activity, DBN-1 is capable of actin bundling. To identify the actin-binding site in DBN-1, we separately analysed the actin-binding properties of the isolated glutathione S -transferase (GST)-fused ADF-H (amino acid (aa) 1–154), coiled-coil (aa 154–368), proline-rich (aa 368–590) and SH3 (aa 590–643) domains ( Fig. 4f ). Under identical experimental conditions, only the coiled-coil domain (aa 154–368) showed significant actin binding. However, actin-binding activities of the ADF-H and proline-rich domains of DBN-1 cannot be excluded to occur under other conditions. We further confirmed the actin-bundling ability of DBN-1 by direct imaging. In the presence of GST-DBN-1, short fluorescently labelled actin filaments assembled into bundles. Surprisingly, longer bundles were often twisted at the ends and shorter ones appeared as rings ( Fig. 5a–c ). Observing bundles at single-molecule resolution by atomic force microscopy showed that most of actin/DBN-1 bundles contained 3–4, and in some cases up to 10 actin filaments in parallel. GST-DBN-1 molecules could be resolved localized along the sides of filaments ( Fig. 5d–h ). 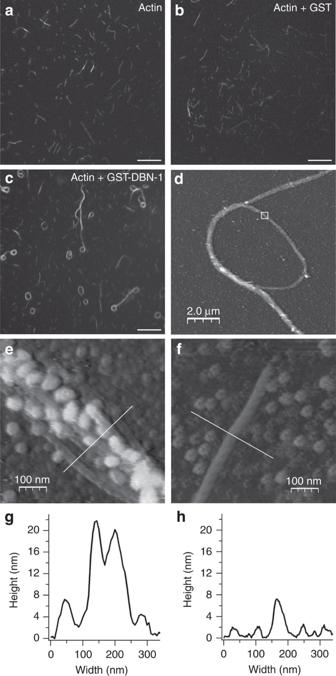Figure 5: Direct visualization of actin filaments bundles generated in the presence of DBN-1. (a) Actin filaments, labelled with rhodamine phalloidin, observed by fluorescence microscopy. (b) Actin filaments in the presence of GST. (c) Bundles of actin filaments formed in the presence of GST-DBN-1 (d) AFM image of a single actin/DBN-1 bundle. (e) High-magnification image of a region of the bundle shown ind. Single molecules of GST-DBN-1 decorated the sides of actin filaments. (f) AFM image of an actin filament in the absence of DBN-1. (g,h) Height profiles along the lines marked ineandf. Figure 5: Direct visualization of actin filaments bundles generated in the presence of DBN-1. ( a ) Actin filaments, labelled with rhodamine phalloidin, observed by fluorescence microscopy. ( b ) Actin filaments in the presence of GST. ( c ) Bundles of actin filaments formed in the presence of GST-DBN-1 ( d ) AFM image of a single actin/DBN-1 bundle. ( e ) High-magnification image of a region of the bundle shown in d . Single molecules of GST-DBN-1 decorated the sides of actin filaments. ( f ) AFM image of an actin filament in the absence of DBN-1. ( g , h ) Height profiles along the lines marked in e and f . Full size image DBN-1 regulates actin filaments during muscle contraction If DBN-1 can bind and bundle actin filaments, what happens to the sarcomere structure on dbn-1 mutation or deletion? We analysed live transgenic worms expressing the tagged actin isoform GFP-ACT-2 in the dbn-1 (ok925) mutant background. The dbn-1 (ok925) has a partial deletion in the K08E3.4 gene, resulting in the expression of truncated DBN-1 (aa 1-301), containing the ADF-H and two coiled-coil domains ( Fig. 6a,b ). In relaxed muscle, actin localization in the dbn-1 (ok925) mutant was indistinguishable from wild type (compared by mean fluorescent intensity variance, n =10, P >0.7, two-tailed Student’s t -test). However, we observed a mild disorganization of actin filaments during muscle contraction in the dbn-1 (ok925) mutant worms, which was nevertheless significant as confirmed by a decrease of the mean fluorescence intensity variance ( n =10, P <0.05, two-tailed Student’s t -test) ( Fig. 6c,d ; Supplementary Movies 2 and 3 ). Since truncated DBN-1 could still interact with F-actin, we additionally analysed worms in which DBN-1 expression was suppressed by RNA-mediated interference (RNAi). We could not detect an aggravation of the actin-disorganization phenotype in dbn-1 (RNAi) worms ( Fig. 6c ; Supplementary Fig. 1a ). These results suggest that DBN-1 is involved in the stabilization of actin filaments in contracted muscle and that a C-terminal part of DBN-1 is involved in this function. 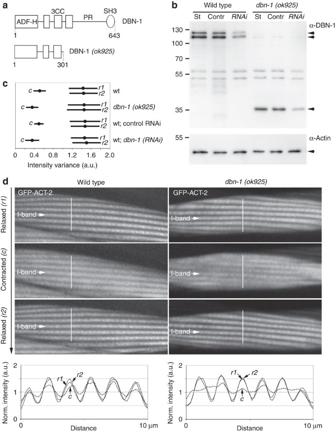Figure 6: Organization of actin filaments (ACT-2) in thedbn-1 (ok925)mutant during contraction. (a) Schematic representation of DBN-1 expressed indbn-1 (ok925)mutant. (b) Western blot analysis of DBN-1 and actin expression in wild-type anddbn-1 (ok925)mutant worms. Total lysates from wild-type ordbn-1 (ok925)worms cultured under standard conditions (St), control RNAi, ordbn-1RNAi were separated by SDS–polyacrylamide gel electrophoresis, transferred onto a polyvinylidene difluoride membrane and stained with anti-DBN-1 antibodies. The same membrane stained with anti-actin antibodies. Molecular mass markers in kDa are indicated on the left. (c) Plots of the fluorescence intensity variances in the relaxed (r1), maximally contracted (c) and again relaxed (r2) state for wild-type worms,dbn-1 (ok925)mutants, wild-type worms treated with control RNAi and wild-type worms treated with RNAi against DBN-1 (n=10 for each condition). The circles represent means, the whiskers are s.d. (d) Localization of GFP-ACT-2 in wild-type and indbn-1 (ok925)mutant worms. Each panel represents images of a body wall muscle cell at the states of relaxation(r1), maximal contraction(c)and again relaxation(r2)during a single contraction cycle. Profiles of normalized fluorescence intensity along the depicted lines. Note the partial disorganization of actin filaments during muscle contraction. Videos of contracting muscles are available in theSupplementary information(Supplementary Movies 2 and 3). Figure 6: Organization of actin filaments (ACT-2) in the dbn-1 (ok925) mutant during contraction. ( a ) Schematic representation of DBN-1 expressed in dbn-1 (ok925) mutant. ( b ) Western blot analysis of DBN-1 and actin expression in wild-type and dbn-1 (ok925) mutant worms. Total lysates from wild-type or dbn-1 (ok925) worms cultured under standard conditions (St), control RNAi, or dbn-1 RNAi were separated by SDS–polyacrylamide gel electrophoresis, transferred onto a polyvinylidene difluoride membrane and stained with anti-DBN-1 antibodies. The same membrane stained with anti-actin antibodies. Molecular mass markers in kDa are indicated on the left. ( c ) Plots of the fluorescence intensity variances in the relaxed ( r1 ), maximally contracted ( c ) and again relaxed ( r2 ) state for wild-type worms, dbn-1 (ok925) mutants, wild-type worms treated with control RNAi and wild-type worms treated with RNAi against DBN-1 ( n =10 for each condition). The circles represent means, the whiskers are s.d. ( d ) Localization of GFP-ACT-2 in wild-type and in dbn-1 (ok925) mutant worms. Each panel represents images of a body wall muscle cell at the states of relaxation (r1) , maximal contraction (c) and again relaxation (r2) during a single contraction cycle. Profiles of normalized fluorescence intensity along the depicted lines. Note the partial disorganization of actin filaments during muscle contraction. Videos of contracting muscles are available in the Supplementary information ( Supplementary Movies 2 and 3 ). Full size image Regulation of ADF/cofilin, tropomyosin and α-actinin In addition to stabilizing actin filaments, DBN-1 might also function to compete other actin-binding proteins away from actin in well-defined locations. This implies, in turn, that in the absence of functional DBN-1, other actin-binding proteins located in close proximity might occupy the vacant binding sites on actin filaments. To test this hypothesis, we examined the localization of GFP-tagged ADF/cofilin (UNC-60B), tropomyosin (LEV-11) and α-actinin (ATN-1) in body wall muscle cells of dbn-1 (ok925) mutant and dbn-1 (RNAi) worms during contraction. UNC-60B is an I-band protein, which controls the turnover of actin filaments by accelerating the rate of depolymerization at the pointed ends and by severing actin filaments [22] , [14] . Fluorescence microscopy of contracting body wall muscles of C. elegans revealed that GFP-UNC-60B was indeed abnormally accumulated along I-bands in the contracted state in the dbn-1 (ok925) mutant and in dbn-1 (RNAi) worms compared with the regular pattern in wild-type worms ( Fig. 7 ; Supplementary Movies 4 and 5 ; Supplementary Fig. 1b ). This observation can explain the partial disorganization of actin at the I-bands in the mutant worms. 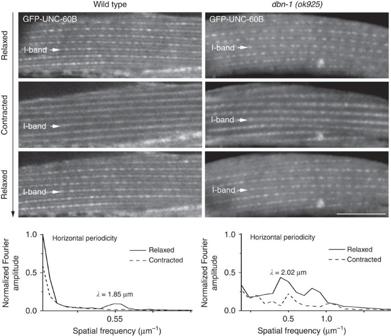Figure 7: Organization of ADF/cofilin (UNC-60B) in thedbn-1 (ok925)mutant during contraction. Localization of GFP-UNC-60B in wild-type and indbn-1 (ok925)mutant worms. Each panel represents images of a body wall muscle cell at the states of relaxation, maximal contraction and again relaxation during a single contraction cycle. Spatial frequency profiles of GFP-UNC-60B pattern in the relaxed (solid line) and contracted (dashed line) state along I-bands. Spatial periods corresponding to the FFT peaks are indicated. Videos of contracting muscles are available in theSupplementary information(Supplementary Movies 4 and 5). Figure 7: Organization of ADF/cofilin (UNC-60B) in the dbn-1 (ok925) mutant during contraction. Localization of GFP-UNC-60B in wild-type and in dbn-1 (ok925) mutant worms. Each panel represents images of a body wall muscle cell at the states of relaxation, maximal contraction and again relaxation during a single contraction cycle. Spatial frequency profiles of GFP-UNC-60B pattern in the relaxed (solid line) and contracted (dashed line) state along I-bands. Spatial periods corresponding to the FFT peaks are indicated. Videos of contracting muscles are available in the Supplementary information ( Supplementary Movies 4 and 5 ). Full size image LEV-11 is bound to actin filaments in the overlap region with myosin, between I-bands and M-lines, showing a clear double-line localization pattern in the body wall muscles of wild-type animals [14] , [34] . In the dbn-1 (ok925) mutants and dbn-1 (RNAi) worms, a significant amount of GFP-LEV-11 appeared at I-bands in relaxed muscles ( Fig. 8a ; Supplementary Movies 6 and 7 ; Supplementary Fig. 2a ). 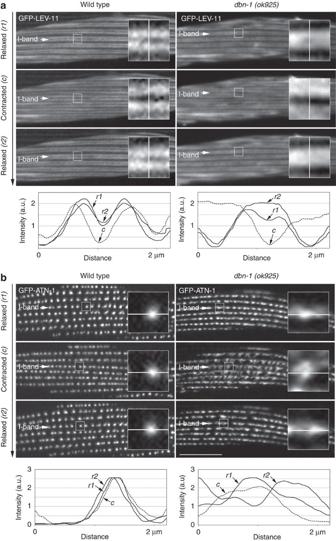Figure 8: Organization of tropomyosin (LEV-11) and α-actinin (ATN-1) in thedbn-1 (ok925)mutant during contraction. (a) Localization of GFP-LEV-11 in wild-type and indbn-1 (ok925)mutant worms. Each panel represents images of a body wall muscle cell in the relaxed state, at maximal contraction and again in the relaxed state during a single contraction cycle. Inserts are zooms of areas outlined by frames. Fluorescence intensity profiles along the lines perpendicular to the I-band marked in the images. Movies of contracting muscles are available in theSupplementary information(Supplementary Movies 6 and 7). (b) Localization of GFP-ATN-1 in wild-type and indbn-1 (ok925)mutant worms in the same contraction states as described ina. Inserts are zooms of areas outlined by frames. Scale bar, 10 μm. Fluorescence intensity profiles along the lines marked in the images. Movies of contracting muscles are available in theSupplementary information(Supplementary Movies 8 and 9). Figure 8: Organization of tropomyosin (LEV-11) and α-actinin (ATN-1) in the dbn-1 (ok925) mutant during contraction. ( a ) Localization of GFP-LEV-11 in wild-type and in dbn-1 (ok925) mutant worms. Each panel represents images of a body wall muscle cell in the relaxed state, at maximal contraction and again in the relaxed state during a single contraction cycle. Inserts are zooms of areas outlined by frames. Fluorescence intensity profiles along the lines perpendicular to the I-band marked in the images. Movies of contracting muscles are available in the Supplementary information ( Supplementary Movies 6 and 7 ). ( b ) Localization of GFP-ATN-1 in wild-type and in dbn-1 (ok925) mutant worms in the same contraction states as described in a . Inserts are zooms of areas outlined by frames. Scale bar, 10 μm. Fluorescence intensity profiles along the lines marked in the images. Movies of contracting muscles are available in the Supplementary information ( Supplementary Movies 8 and 9 ). Full size image ATN-1 is normally localized on the cytoplasmic side of dense bodies [11] . A regular organization of GFP-ATN-1 is retained during muscle contraction and relaxation in wild-type worms ( Fig. 8b ; Supplementary Movie 8 ). Mutation in dbn-1 , or treatment of worms with RNAi against DBN-1, in contrast, resulted in irregular patterns of α-actinin accumulations already in the relaxed state which became even more dramatic during contraction ( Fig. 8b ; Supplementary Movie 9 ; Supplementary Fig. 2b ). Taken together, these data suggest that DBN-1’s function in sarcomeres includes a protective role that is important for the proper localization of ADF/cofilin, tropomyosin and α-actinin along actin filaments. Sequence analysis showed that DBN-1 (DreBriN 1/DreBriN-like homologue) is a C. elegans member of the drebrin/Abp1 class of ADF-H proteins. Our experiments have clearly demonstrated that DBN-1 is involved in sarcomere organization and function. DBN-1 mediates proper spacing of α-actinin and tropomyosin and stabilizes actin filaments during muscle contraction, possibly strengthening them by bundling. The presence of the SH3 domain in the primary structure of DBN-1 indicates that this protein is a C. elegans Abp1 (refs 33 , 35 ). Nevertheless, the C. elegans genome does not encode an independent drebrin 1 gene, and thus DBN-1 could represent a ‘hybrid’ or developmental progenitor of two proteins, mAbp1 and drebrin. Indeed, the proline-rich domain of DBN-1 shows more sequence similarity to drebrin than to mAbp1. In contrast to both proteins, DBN-1 has three isolated coiled-coil domains, and thus could also be classified as an independent member of the drebrin/Abp1 class. We have shown that DBN-1 binds to actin filaments and bundles them in vitro . Actin binding occurs with moderate affinity ( K d =4.1±0.3 μM), that is more similar to mAbp1 ( K d =2.2±0.5 μM) [33] than to drebrin ( K d =0.12 μM) [36] . The stoichiometry of actin binding was ∼ 1 molecule of His-DBN-1 to 18–19 molecules of actin in contrast to 1:5 for mAbp1 (ref. 33 ) and drebrin [36] . Under our experimental conditions, only the coiled-coil domain (aa 154–368) clearly showed actin-binding activity; the interaction of ADF-H and proline-rich domains with actin cannot be excluded under other conditions. In addition to actin binding, DBN-1 is also able to bundle actin filaments. Interestingly, a cryptic actin-bundling activity of drebrin has been recently described [37] . The actin-bundling activity of DBN-1 is most likely mediated by the presence of the three isolated coiled-coil domains adjoining the ADF-H domain. It is tempting to speculate that in vivo DBN-1 bundles neighbouring actin filaments of the same sarcomere and/or filaments of the adjacent sarcomeres between dense bodies, thus strengthening them during contraction. DBN-1 inside the sarcomere re-localized dynamically from M-lines at relaxation to I-bands at contraction. Partial co-localization of DBN-1 with ATN-1 suggests that DBN-1 might directly interact with α-actinin or other proteins, located in close proximity at dense bodies. For example, DBN-1 is a possible target for phosphorylation by Src-1 (ref. 38 ). Association of DBN-1 and LEV-11 with distinct parts of actin filaments at muscle contraction suggests that DBN-1 and tropomyosin compete for the binding to F-actin. This notion is consistent with the reported competition between mammalian drebrin and other actin-binding proteins, such as tropomyosin, α-actinin and myosin for actin filaments in vitro and in cultured fibroblast [36] , [39] , [40] . DBN-1 loss of function resulted in the partial disorganization of actin filaments at I-bands during muscle contraction in vivo . This observation is in agreement with the finding that drebrin protects F-actin from depolymerization in vitro [41] . Destabilization of actin filaments in the contracted state in dbn-1 (ok925) mutants or under dbn-1 (RNAi) occurs likely due to increased access of UNC-60B to actin filaments. This effect was not very marked, however, possibly due to the tendency of other actin-binding proteins with actin-stabilizing properties to bind vacant sites on actin filaments. Indeed, we found that α-actinin and tropomyosin in dbn-1 (ok925) and dbn-1 (RNAi) worms were displaced to the sites where DBN-1 is normally present. In addition, compensatory stabilization of actin filaments can be provided by kettin [34] and titin [42] . As a recurring theme in biology where multi-protein machineries such as the centrosome or focal adhesions depend on a large number of different players, DBN-1 appears to be part of a subtly balanced assembly of actin stabilizers tailored to keep the muscle machinery dynamically organized during muscle contraction cycles. It is apparent, however, that this role of DBN-1 is not its only one. On the basis of the intracellular localization of DBN-1 and on a tentative functional comparison with its relatives, DBN-1 could furthermore modulate the plasticity and function of postsynaptic sites of neuromuscular junctions, analogous to mAbp1 and drebrin, which are known as essential players in both neurological [43] , [44] , [45] , [28] and immunological [30] , [29] synapses. In addition, DBN-1 may be involved in vesicle transport, similar to yeast and mammalian Abp1 homologues, which are well-described key regulators of receptor-mediated endocytosis, vesicle trafficking and endocytic structure disassembly [46] , [47] , [48] , [49] , [32] . The recent identification of mAbp1 as an adaptor protein linking β-integrin family molecules to the actin cytoskeleton [50] indicates a possible function of DBN-1 in signalling pathways from the extracellular environment via integrin-based dense bodies and M-lines to the sarcomeres. Close association of DBN-1 with the SCA-1 both during contraction and relaxation, suggests a potential role of DBN-1 in mediating excitation–contraction coupling, similar to drebrin, which has been identified as a regulator of calcium response [51] . In addition, the generation and analysis of mAbp1-knockout mice produced unambiguous data that implicate this gene in the formation of hypertrophic cardiomyopathy [32] . Therefore, C. elegans should prove an excellent model system to understand the up to now unknown functions of the drebrin/Abp1 class of proteins in muscle cells. C. elegans strains C. elegans strains were cultured at 20 °C using the standard protocols [52] . The wild-type Bristol N2 and ok925 strains were obtained from the C. elegans Genetic Center (University of Minnesota). Expression constructs To generate a dbn-1 promoter-GFP construct, a 2,003 bp DNA fragment upstream of the K08E3.4 coding sequence was amplified by PCR from wild-type C. elegans genomic DNA and cloned into prab-3::GFP (kindly provided by Stefan Eimer, University of Freiburg) between SphI and BamHI to replace the rab-3 promoter. Dbn-1 , act-2, unc-60B, lev-11, atn-1, sca-1 and myo-3 coding sequences were amplified by PCR from C. elegans complementary DNA, subcloned into pDonr 201 vector (Invitrogen) and subsequently cloned into Gateway destination vectors phim-4::GFP-Gateway , phim-4::mCherry-Gateway or pmyo-3::GFP-Gateway. To construct GST-dbn-1 and His-dbn-1 , DNA sequence, encoding the full-length DBN-1 (aa 1–643), was cloned between BamHI and XhoI sites of the pGEX 4T3 vector or BamHI and SalI sites of the pET28a vector, respectively. DNA sequences, encoding for the ADF-H (aa 1–154), coiled-coil (aa 154–368), proline-rich (aa 368–590) and SH3 (aa 590–643) domains were cloned between the BamHI and SalI sites of the pGEX 4T3 vector. To generate BiFC constructs, act-2 and dbn-1 coding sequence were cloned into pCMV-VN155-Gateway and pCMV-VC155-Gateway , respectively. Transgene generation and crossings Transgenic strains were generated by microinjection [53] of the plasmids phim-4::mCherry-dbn-1 , phim-4::mCherry-atn-1 , phim-4::mCherry-sca-1 , phim-4::mCherry-myo-3 , phim-4::GFP-dbn-1 , pmyo-3::GFP-act-2 , phim-4::GFP-lev-11 , phim-4::GFP-atn-1 and phim-4::GFP-unc-60B at 5–20 ng μl −1 alone or in combination. pRF4 (rol-6(su1006)) (100 ng μl −1 ) and pRFP-odr-1 (50 ng μl −1 ) were used as co-injection markers. Crossings of Ex [myo-3::GFP-ACT-2], Ex [him-4::GFP-UNC-60B], Ex [him-4::GFP-LEV-11] and Ex [him-4::GFP-ATN-1] with dbn-1 (ok 925) were performed using classical genetic approaches. C. elegans cell culture Muscle cells were isolated from L2–L4 larvae as described in ref. 54 . Isolated cells were grown in L-15 medium (Invitrogen) supplemented with 10% fetal bovine serum (Invitrogen), 50 U ml −1 penicillin and 50 μg ml −1 streptomycin (Sigma-Aldrich) on coverslips coated with 0.5 mg ml −1 peanut lectin (Sigma-Aldrich) at 20 °C. Live cells were analysed by fluorescence microscopy 30 h after plating. Mammalian cell culture and transfection COS-7 cells were obtained from the DSMZ (Leibniz Institute DSMZ-German Collection of Microorganisms and Cell Cultures, Braunschweig, Germany) and cultured in DMEM supplemented with 10% FCS, 100 U ml −1 penicillin and 100 μg ml −1 streptomycin (Sigma-Aldrich) in a humidified 5% CO 2 atmosphere at 37 °C. Transient transfection was performed by electroporation using Lonza nucleofector. pCMV-VN155-ACT-2 and pCMV-VC155 ; pCMV-VC155-DBN-1 and pCMV-VN155 ; pCMV-VN155-ACT-2 and pCMV-VC155-DBN-1 were co-transfected. Cells were fixed with 4% paraformaldehyde in PBS 24 h after transfection and the BiFC signal was analysed by fluorescence microscopy. Protein electrophoresis and western blot Fifty young adult worms were lysed in 20 μl of nematode solubilization buffer (2 mM EDTA, 5 mM DTT, 0.3% ethanol amine in M9 buffer). Then 20 μl of 2 × Laemmli buffer was added and the sample was heated to 95 °C for 2 min, homogenized by brief sonication and heated again to 95 °C for 2 min. Ten microlitre of sample were resolved by SDS–PAGE using a 12% acrylamide gel. Proteins were transferred onto a polyvinylidene difluoride membrane (Immobilon-P; Millipore, Billerica, MA, USA) using a Bio-Rad Criterion Blotter. The membrane was blocked with 10% non-fat milk in PBS containing 0.05% Tween 20 for 30 min and incubated with affinity-purified anti-DBN-1 antibodies diluted at 1:500 at 4 °C overnight, followed by treatment with peroxidase-labelled goat anti-Rabbit IgG (A6154, Sigma-Aldrich). The reactivity was detected with an Amersham ECL Detection Reagent (GE Healthcare Life science) using an Intas gel imager (Intas Science Imaging Instruments GmbH). The membrane was treated with a buffer containing 2% SDS, 100 mM β-mercaptoethanol, and 62.5 mM Tris-HCl, pH 6.8, at 50 °C for 30 min to remove bound probes and reprobed with mouse monoclonal anti-actin antibody (clone C4; MP Biomedicals) in combination with peroxidase-labelled goat anti-mouse IgG (A6154, Sigma-Aldrich). RNA interference experiments The dbn-1 complementary DNA fragment corresponding to positions 1–500 bp was amplified by PCR and cloned into the L4440 feeding vector [55] between Nhe I and Kpn I sites. E. coli HT115 (DE3), an RNase III-deficient strain [56] , was transformed with the L4440 vector containing this 500 bp dbn-1 fragment. Control experiments were performed with the HT115 (DE3) that was transformed with an empty L4440 vector. RNAi was performed as described [14] . Briefly, the transformed bacteria were cultured overnight at 37 °C in LB containing 50 μg ml −1 ampicillin, applied onto 6-cm plates containing NGM agar with 1 mM isopropyl-β- D -thiogalactoside and 25 μg ml −1 carbenicillin, and incubated overnight at room temperature. Ten wild-type worms at the L4 stage were transferred onto the plates and allowed to lay eggs during 24 h at 20 °C. F1 were cultured at 20 °C, and phenotypes were analysed at their young adult stage. Production of antibodies Recombinant full-length DBN-1 was used to immunize two rabbits at Bioscience (Göttingen, Germany). The antiserum from both rabbits was purified using NHS-activated Sepharose High Performance (GE Healthcare Life Science). Immunohistochemistry Worms were fixed and permeabilized according to Bouin’s tube fixation protocol ( www.wormbook.com ). Affinity-purified anti-DBN-1 antibodies (1:500) were used in combination with Alexa Fluor 488-labelled goat anti-rabbit IgG (A11008; Molecular Probes; 1:1,000). Commercial monoclonal antibodies against actin (clone C4; MP Biomedicals; 1:500) were used in combination with fluorescein isothiocyanate-labelled goat anti-mouse IgG (F0257; Sigma; 1:1,000). Fluorescence microscopy Young adult-stage worms were treated with 5 mM tetramisole for 1–3 min or with 10 mM muscimol for 20–25 min until paralysed and mounted on 4% agarose pads. To observe contracting muscles, microscope slides were modified by introducing walls to create a gap between agarose layer and cover slip. In such chambers, worms were anchored without compression. The muscle contractions were recorded during the first 3 min after placing the worms in M9 buffer in such a chamber. Fluorescence images were obtained using an Axiovert 200M microscope equipped with both a 63 × /numerical aperture (NA) 1.4 and 40 × /NA 1.3 objective, a spinning disk confocal unit (Yokagawa CSU10) and an Andor iXon EM-CCD camera. Quantification of fluorescent intensity variance To quantify the variance of fluorescence intensity of GFP-ACT-2, time-lapse images were recorded, always with the same acquisition parameters (200-ms exposure time and a readout time between frames of 44 ms). Single frames, corresponding to maximally relaxed, maximally contracted and again maximally relaxed states of the same contraction cycle of 10 different muscles ( n =10) for each condition (wild type, dbn-1 (ok925) , control RNAi and dbn-1 (RNAi) ) were extracted. Images were filtered using an ImageJ variance radius 2-pixel filter. The raw integrated density was measured within a 10 × 10 μm frame drawn in the middle of the muscle. Means and s.d. values were calculated for each condition and plotted on a graph. The data were tested for a normal distribution. The group data for each individual condition were compared using a two-tailed Student’s t -test. Values of P <0.05 were considered statistically significant. Fourier analysis of fluorescence images To quantify the spatial frequency of the striated patterns in the fluorescence images, rectangular sections of ∼ 10 × 20 μm were cut out and Fourier transformed. These two-dimensional Fast Fourier transformations (FFTs) were carried out with the WSxM software (Nanotec, Madrid, Spain) and ImageJ software. The two-dimensional FFT images were averaged in the direction perpendicular to the frequency pattern to obtain the one-dimensional spatial frequency profiles that are presented in the images. Expression and purification of recombinant proteins Recombinant proteins were expressed in E. coli XL1 blue cells at 24 °C in the presence of 100 μM isopropyl-β- D -thiogalactoside. His-DBN-1was purified on Ni-NTA Agarose (Macherey-Nagel); GST-DBN-1 and its domain constructs were purified on Glutathione Sepharose 4 Fast Flow beads (GE Healthcare) according to the manufacturer’s protocol. In vitro F-actin co-sedimentation assay F-actin was prepared from rabbit muscle acetone powder as described in the literature [57] , [58] , and suspended in 0.1 M KCl, 20 mM imidazole, pH 7.0 at a concentration of 5 mg ml −1 . To calculate the molar concentration of proteins, the molecular masses 42 kDa for actin and 75 kDa for His-DBN-1 were used. The actin-binding assay was performed using increasing His-DBN-1 concentrations (0.13, 0.15, 0.21, 0.32, 0.43 and 0.64 μM) and a constant actin concentration (0.7 μM). His-DBN-1 was incubated with F-actin in F-buffer (2 mM HEPES, 2 mM MgCl 2 , 0.05 mM KCl, 1 mM Na 2 ATP, 1 mM EGTA) at room temperature for 1 h. Then, the reaction mixtures were centrifuged in an Airfuge (Beckman Instruments) at 100,000 g for 30 min. Actin-binding assays with GST-tagged ADF-H, 3CC, PR and SH3 domains were performed under the same conditions. For the actin-bundling assay, 1.4 μM F-actin and 0.21 μM His-DBN-1 alone or together were incubated in F-buffer at room temperature for 1 h and centrifuged at 10,000 g for 30 min. After centrifugation, supernatants and pellets were adjusted to the same volumes and proteins were separated by 12% SDS–PAGE followed by staining with Page Blue protein staining solution (Thermo Scientific). Gels were scanned using an Intas gel imager (Intas Science Imaging Instruments GmbH), and intensities of protein bands were analysed using ImageJ Software ( http://imagej.nih.gov/ij , v1.48t). The dissociation constant K d for binding of His-DBN-1 to actin was determined by quantification of the actin-bound/unbound protein fraction, f as a function of the concentration of actin A and the concentration of DBN-1 DBN . Data were fit by the following equation with Origin 8.5ProG (Origin Labs Corp, Northampton, MA, USA): Actin labelling and actin-DBN-1 interaction in vitro Ten microlitre of actin (5 mg ml −1 ) were polymerized at room temperature in 10 × F-buffer for 30 min. Three hundred units of rhodamine phalloidin (R415, Invitrogen) were dissolved in 1.5 ml of methanol. To label actin, 4 μl of rhodamine phalloidin was mixed with 3 μl of polymerized actin in 93 μl of F-buffer (2 mM HEPES, 2 mM MgCl 2 , 0.05 mM KCl, 1 mM Na 2 ATP, 1 mM EGTA). The labelled actin was then diluted 1:50 in AB buffer (2 mM MgCl 2 , 1 mM ATP, 10 mM DTT, 0.1 mg ml −1 glucose-oxidase, 0.018 mg ml −1 catalase and 2.3 mg ml −1 glucose in F-buffer). Glass chambers were filled with 10 μl of GST-DBN-1 (0.8 mg ml −1 ) or GST alone (0.5 mg ml −1 ) and incubated for 5–10 min. Then, 10 μl of labelled actin in AB buffer were added into these or empty chambers. Fluorescence microscopy pictures were recorded after 5–20 min using the NA 1.3 objective. For atomic force microscope (AFM) imaging, 10 μl of labelled actin or 10 μl of GST-DBN-1 and 10 μl of labelled actin in AB buffer were applied to a glass coverslip coated with a positively charged silane (3-[2-(2-aminoethylamino) ethylamino] propyltrimethoxysilane (Sigma-Aldrich), and actin filament bundles were allowed to attach to the surface for 5 min. Then, 150 μl of AB buffer was added to prevent sample drying. AFM and cantilevers AFM imaging was carried out on a MFP-3D (Asylum Research, Santa Barbara, CA) using Olympus BL-RC150VB cantilevers (30 × 50 μm, spring constant≈0.03 N m −1 , tip radius≈30 nm, Olympus, Tokyo, Japan). The images of actin filaments were acquired using tapping mode [59] (oscillating the cantilever at≈4 kHz with a 3-nm amplitude), and the estimated force applied to the sample was <0.1 nN. How to cite this article: Butkevich, E. et al . Drebrin-like protein DBN-1 is a sarcomere component that stabilizes actin filaments during muscle contraction. Nat. Commun. 6:7523 doi: 10.1038/ncomms8523 (2015).